UHRF1 targets DNMT1 for DNA methylation through cooperative binding of hemi-methylated DNA and methylated H3K9 Epigenetic inheritance of DNA methylation in mammals requires a multifunctional protein UHRF1, which is believed to recruit DNMT1 to DNA replication forks through a unique hemi-methylated CpG-binding activity. Here we demonstrate that the UHRF1 mutants deficient in binding either hemi-methylated CpG or H3K9me2/3, but not both, are able to associate with pericentric heterochromatin, recruit Dnmt1 and partially rescue DNA methylation defects in mouse Uhrf1 null ES cells. Furthermore, we present evidence that the flip out of the methylated cytosine induced by UHRF1 binding is unlikely essential for subsequent DNA methylation by DNMT1. Together, our study demonstrates that UHRF1 can target DNMT1 for DNA maintenance methylation through binding either H3K9me2/3 or hemi-methylated CpG, and that the presence of both binding activities ensures high fidelity DNA maintenance methylation. In addition, our study indicates that UHRF1 mediates cross-talk between H3K9 methylation and DNA methylation at the level of DNA methylation maintenance. In mammals, DNA methylation predominantly occurs at cytosine-C5 in the context of CpG dinucleotides [1] . DNA methylation is established and maintained by three active DNA methyltransferases, DNMT3a, DNMT3b and DNMT1 [2] , [3] . Both DNMT3a and DNMT3b have de novo DNA methylation activity, whereas DNMT1 has a strong preference for hemi-methylated CpG (mCpG) substrates generated during DNA replication and has a central role in maintaining the patterns of DNA methylation through cell division [2] , [3] , [4] . Cumulative studies provide compelling evidence for critical roles of DNA methylation in transcriptional regulation, heterochromatin formation, X-inactivation, imprinting and genome stability. Aberrant DNA methylation is associated with pathological processes including cancer [5] , [6] . Consistent with its central role in DNA maintenance methylation, DNMT1 is associated with DNA replication forks in the S phase of cell cycle [7] , [8] . How DNMT1 is recruited to the DNA replication foci has been a central topic for study. DNMT1 was shown to interact with proliferating-cell nuclear antigen (PCNA), a cofactor of DNA polymerase delta and component of the DNA replication forks [9] . However, subsequent studies indicated that PCNA is insufficient to recruit DNMT1 [10] , [11] and identified UHRF1 (also known as ICBP90 in human and NP95 in mouse) as a DNMT1-interacting protein essential for targeting DNMT1 to replication forks and DNA maintenance methylation [12] , [13] . UHRF1 is a multi-structural and functional nuclear protein [12] , [13] , [14] , [15] , [16] , [17] . It contains a unique SET and ring-associated domain (SRA) domain that recognizes preferentially hemi-mCpG, the product of newly replicated DNA. The binding of hemi-mCpG by SRA involves a novel 5-methylcytosine (5-mC) flip out mechanism that is also observed for DNA methyltransferases [18] , [19] , [20] . This observation has led to the idea that the flip out of the pre-existing methylated cytosine is associated with the coordinated transfer of the hemi-mCpG site from UHRF1 to DNMT1. In addition, UHRF1 also possesses an H3K9me2/3-specific-binding activity and has been shown to associate with pericentric heterochromatin [21] , [22] , [23] , [24] , [25] . However, the exact function of the hemi-mCpG and H3K9me2/3 binding activities in targeting DNMT1 to replication forks and maintenance methylation is not clear. Here we have systematically studied the role of UHRF1 hemi-mCpG and H3K9me2/3-binding activities in its heterochromatin association, targeting DNMT1 to DNA replication foci and DNA methylation maintenance. We present evidence that the flip out of the methylated cytosine by UHRF1 binding is unlikely essential for subsequent DNA methylation by DNMT1. UHRF1 mutants deficient in binding of H3K9me2/3 or hemi-mCpG Using a series of UHRF1 deletion mutants and in vitro peptide pulldown assay, we mapped the H3K9me2/3-binding activity to the region of a tandem tudor domain (Tudor)/a plant homeodomain (PHD) ( Fig. 1a ). Disruption of Tudor domain (mutant aa182-408) led to loss of H3K9me2/3-binding specificity, whereas the deletion of PHD domain maintained the H3K9me2/3-binding specificity but reduced substantially the binding activity ( Fig. 1a ). These results indicate that the Tudor domain is responsible for H3K9me2/3-binding specificity and that the PHD domain contributes to the overall binding activity, in agreement with the reported structural studies [22] , [23] , [24] , [25] . The structural study indicates that within Tudor domain Tyr191 directly interacts with the K9me3, whereas Trp238 is involved in the formation of H3 peptide binding pocket [25] . Consistently, we found two mutants, one with Tyr191 and Pro192 changed to Ala (YP191/192AA) and the other with Phe237 and Trp238 to Ala (FW237/238AA) were defective in binding of H3K9me2 ( Fig. 1b ). As expected, these mutants maintain the hemi-mCpG-binding activity in gel mobility shift assay ( Supplementary Fig. S1a ). 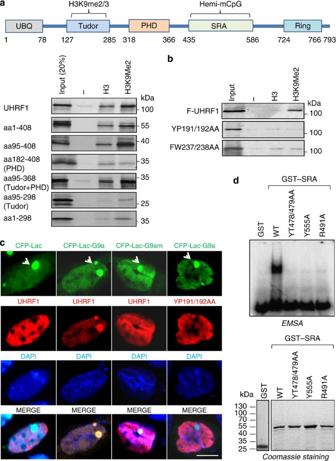Figure 1: Characterization of UHRF1 mutants defective in binding either H3K9me2/3 or hemi-mCpG. (a) Diagram illustrating the structural organization of UHRF1 protein. The relative position of each domain is indicated by the number. Pulldown was performed within vitrosynthesized and 35S-met labelled UHRF1 proteins and control H3 tail peptide (aa1-21) and H3K9me2 peptide (aa1-21). The binding of various UHRF1 proteins was revealed by autoradiography. UBL, ubiquitin-like domain; Ring, really interested new gene domain. (b) The UHRF1 Tudor mutants were synthesized as above and tested for binding of H3K9me2 peptide byin vitropulldown. (c) The UHRF1 and Tudor mutants were tested forin vivoH3K9me2/3-binding activity in CHO DG44 cells. The CHO DG44 cells were transfected with control CFP-Lac, CFP-Lac-G9a or CFP-Lac-G9am (H1113K enzymatic defective mutant), together with Flag-UHRF1 or Flag-UHRF1 mutants as indicated. The cells were then processed for immunofluoresence analysis for UHRF1 and mutants using anti-Flag antibody and co-localization with CFP-Lac or CFP-Lac-G9a fusion proteins was analysed. The arrow indicates the lac operon locus bound by CFP-Lac or CFP-Lac-fusions of G9a or G9am. Scale bar, 5 μm. (d) Gel mobility shift assay with hemi-methylated DNA probe and UHRF1 SRA mutants. The hemi-mCpG duplex was labelled with 32p-dCTP using klenow fragment. Lower panel shows Coomassie blue staining gel of the recombinant proteins used for gel mobility shift assay. Figure 1: Characterization of UHRF1 mutants defective in binding either H3K9me2/3 or hemi-mCpG. ( a ) Diagram illustrating the structural organization of UHRF1 protein. The relative position of each domain is indicated by the number. Pulldown was performed with in vitro synthesized and 35S-met labelled UHRF1 proteins and control H3 tail peptide (aa1-21) and H3K9me2 peptide (aa1-21). The binding of various UHRF1 proteins was revealed by autoradiography. UBL, ubiquitin-like domain; Ring, really interested new gene domain. ( b ) The UHRF1 Tudor mutants were synthesized as above and tested for binding of H3K9me2 peptide by in vitro pulldown. ( c ) The UHRF1 and Tudor mutants were tested for in vivo H3K9me2/3-binding activity in CHO DG44 cells. The CHO DG44 cells were transfected with control CFP-Lac, CFP-Lac-G9a or CFP-Lac-G9am (H1113K enzymatic defective mutant), together with Flag-UHRF1 or Flag-UHRF1 mutants as indicated. The cells were then processed for immunofluoresence analysis for UHRF1 and mutants using anti-Flag antibody and co-localization with CFP-Lac or CFP-Lac-G9a fusion proteins was analysed. The arrow indicates the lac operon locus bound by CFP-Lac or CFP-Lac-fusions of G9a or G9am. Scale bar, 5 μm. ( d ) Gel mobility shift assay with hemi-methylated DNA probe and UHRF1 SRA mutants. The hemi-mCpG duplex was labelled with 32p-dCTP using klenow fragment. Lower panel shows Coomassie blue staining gel of the recombinant proteins used for gel mobility shift assay. Full size image Despite strong in vitro biochemical and structural evidence and observed UHRF1 pericentromeric heterochromatin localization [21] , [22] , [24] , [25] , [26] , the H3K9me2/3-binding activity of UHRF1 has not been clearly demonstrated in vivo . To test the H3K9me2/3-binding activity of UHRF1 in vivo , we made use of a CHO cell line, which contains a large number of Lac operator sequences stably integrated in a single chromosomal site [27] . Expression of control CFP-tagged Lac proteins or CFP-Lac fused with H3K9 methyltransferase G9a in these cells generated a bright foci due to the binding of CFP-Lac and CFP-Lac-G9a proteins to the integrated Lac sequences. The expression of CFP-Lac-G9a also resulted in the increased levels of H3K9me3 in the foci ( Supplementary Fig. S2 ). We observed co-localization of ectopically expressed UHRF1 with CFP-Lac-G9a in ~61% cells but none with the control CFP-Lac. Furthermore, the rate of co-localization between UHRF1 and a CFP-Lac-G9a mutant deficient in H3K9 HMT activity [28] dropped drastically to only ~13% ( Fig. 1c ). Similarly, we observed a G9a-enzymatic-activity-dependent co-localization of HP1α, a well-characterized H3K9me2/3-binding protein [29] , [30] , [31] , with CFP-Lac-G9a ( Supplementary Fig. S3 ). In contrast to the wild-type UHRF1, the co-localization of YP191/192AA mutant with the CFP-Lac-G9a foci was observed only in ~7% cells ( Fig. 1c ) and a similar result were observed for FW237/238AA mutants ( Supplementary Fig. S4 ). Together, these results provide compelling evidence that UHRF1 binds H3K9me2/3 in cells and that both YP191/192AA and FW237/238AA mutants are deficient in binding H3K9me2/3. To generate UHRF1 mutants that were deficient in binding of hemi-mCpG, we first made several SRA domain mutants based on the reported SRA–DNA structures. In the SRA binding pocket for hemi-mCpG, Tyr478 interacts with the mC by stacking interaction, whereas Thr479 interacts with the mC by a hydrogen bond [19] . The Arg491 is important for mC flip out as it interrogates the original mC space and forms multiple interactions with the orphaned guanosine [19] . We tested the effect of these mutations on binding of hemi-mCpG using recombinant glutathione S -transferase (GST)–SRA fusion proteins. As shown in Fig. 1d , the YT478/479AA and R491A mutations all abolished the hemi-mCpG-binding activity. Similarly, we found that the Y555A mutant was also defective in binding hemi-mCpG. Furthermore, the same mutations also abolished the hemi-mCpG-binding activity of the full-length UHRF1 ( Supplementary Fig. S1a ). However, these mutations maintained the H3K9me2-binding activity ( Supplementary Fig. S1b ), in agreement with the notion that the H3K9me2/3-binding activity resides in the Tudor/PHD domain. The SRA and Tudor mutants in heterochromatin association UHRF1 has been observed to associate with pericentromeric heterochromatin in both human and mouse cells [21] , [26] , [32] and this property has been linked to its role in DNA methylation [13] . However, it has been controversial whether this association is dependent on its hemi-mCpG or/and H3K9me2/3 binding activities [33] . To address this issue, we expressed various UHRF1 mutants in NIH3T3 cells, whose pericentric heterochromatin can be conveniently visualized as densely stained 4,6-diamidino-2-phenylindole (DAPI) foci, and quantified their co-localization with DAPI foci and H3K9me3. We observed that in ~84% UHRF1-expressing cells Flag-UHRF1 exhibited a focal staining pattern that is overlapped with DAPI foci and H3K9me3 ( Fig. 2a ), whereas in ~16% cells Flag-UHRF1 displayed a diffuse nuclear staining (data not shown). For two Tudor mutants (YP191/192AA and FW237/238AA), the co-localization with DAPI foci ( Fig. 2b ) and H3K9me3 ( Supplementary Fig. S5 ) were observed but at a reduced ratio (56.7% and 41.7%, respectively). For three SRA mutants (YT478/479AA, R491A and Y555A), the co-localization with DAPI foci ( Fig. 2c ) and H3K9me3 ( Supplementary Fig. S5 ) were 33.2%, 35.6% and 36.1%, respectively. Thus, loss of either H3K9me2/3 or hemi-mCpG-binding activity only partially affects the UHRF1 pericentric heterochromatin association. To confirm this observation, we generated two UHRF1 mutants with mutations in both Tudor and SRA domains (YP191/192AA+YT478/479AA and FW237/238+Y555A). Unlike the aforementioned Tudor or SRA mutants, these SRA/Tudor double mutants essentially lost heterochromatin association (4.5% for YP191/192AA+YT478/479AA and 2.1% for FW237/238AA+Y555A). In fact, the double Tudor/SRA mutants exhibited two different staining patterns in NIH3T3 cells, a diffuse nuclear staining pattern in nearly 50% cells and the large focal staining pattern that overlaps neither with the DAPI foci ( Fig. 2d ) nor the nucleolar protein NPM1 ( Supplementary Fig. S6 ) in other 50% cells. When analysed in mouse Uhrf1−/− ES cells, we found that the double Tudor/SRA mutant displays no co-localization with DAPI foci but a diffuse nuclear staining devoid of nucleolus, whereas the wild-type UHRF1 co-localizes with the DAPI foci in ~85% cells ( Fig. 2e ). We thereby conclude that both hemi-mCpG and H3K9me2/3 binding activities have a role in targeting UHRF1 to pericentric heterochromatin regions. 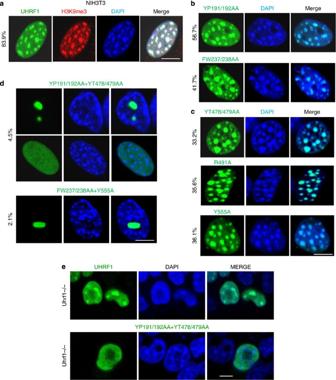Figure 2: UHRF1 associates with pericentric heterochromatin by binding hemi-mCpG and/or H3K9me2/3. (a) The subcellular localization of UHRF1 in NIH3T3 cells were examined by immunostaining. The cells were double immunostained for Flag-UHRF1 (green) and H3K9me3 (white) and costained with DAPI for DNA. The co-localization of UHRF1 with H3K9me3 and densely DAPI-stained pericentric heterochromatin regions was scored in ~83.9% UHRF1-expressing cells. The co-localization of each type of UHRF1 mutants with densely DAPI-stained pericentric heterochromatin regions in NIH3T3 cells was examined by counting more than 300 cells in three independent experiments and the representative results and percentage of co-localization were shown for (b) the Tudor mutants defective in binding H3K9me2/3; (c) the SRA mutants defective in binding hemi-methylated DNA and (d) the double mutants defective in binding both hemi-mCpG and H3K9me2/3. Note only the double mutants nearly completely lost the co-localization with densely DAPI-stained pericentric heterochromatin regions. Scale bar, 5 μm. (e) The wild-type UHRF1 and the YP191/192AA+YT478/479AA Tudor/SRA double mutant were expressed in Uhrf1−/− ES cells and the subcellular localization was revealed by immunostaining using anti-Flag antibody. Scale bar, 5 μm. Figure 2: UHRF1 associates with pericentric heterochromatin by binding hemi-mCpG and/or H3K9me2/3. ( a ) The subcellular localization of UHRF1 in NIH3T3 cells were examined by immunostaining. The cells were double immunostained for Flag-UHRF1 (green) and H3K9me3 (white) and costained with DAPI for DNA. The co-localization of UHRF1 with H3K9me3 and densely DAPI-stained pericentric heterochromatin regions was scored in ~83.9% UHRF1-expressing cells. The co-localization of each type of UHRF1 mutants with densely DAPI-stained pericentric heterochromatin regions in NIH3T3 cells was examined by counting more than 300 cells in three independent experiments and the representative results and percentage of co-localization were shown for ( b ) the Tudor mutants defective in binding H3K9me2/3; ( c ) the SRA mutants defective in binding hemi-methylated DNA and ( d ) the double mutants defective in binding both hemi-mCpG and H3K9me2/3. Note only the double mutants nearly completely lost the co-localization with densely DAPI-stained pericentric heterochromatin regions. Scale bar, 5 μm. ( e ) The wild-type UHRF1 and the YP191/192AA+YT478/479AA Tudor/SRA double mutant were expressed in Uhrf1−/− ES cells and the subcellular localization was revealed by immunostaining using anti-Flag antibody. Scale bar, 5 μm. Full size image Rescue of DNA methylation by Tudor or SRA mutants We next examined the function of the UHRF1 and various mutants in DNA methylation by testing their ability to rescue DNA methylation defect in Uhrf1−/− ES cells. As expected, immunostaining using an anti-5-mC antibody revealed that DNA methylation in Uhrf1−/− ES cells is substantially lower than that in the wild-type E14 ES cells ( Fig. 3a ). Expression of Flag-tagged UHRF1 in Uhrf1−/− ES cells restored the DNA methylation to the wild-type E14 levels ( Fig. 3b , upper panel). Similarly, we found that both Tudor mutants YP191/192AA and FW237/238AA were able to rescue the DNA methylation in Uhrf1−/− ES cells. Notably, we observed that expression of three SRA mutants (YT478/479AA, R491A and Y555A) defective in binding of hemi-mCpG all led to substantial increase of DNA methylation in the Uhrf1−/− ES cells ( Fig. 3b ), indicating that hemi-mCpG-binding activity is also not absolutely required for UHRF1-mediated DNA methylation. 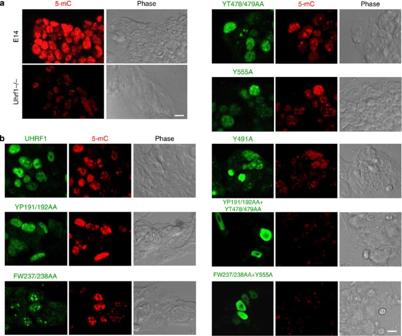Figure 3: Rescue of DNA methylation in Uhrf1−/− ES cells by ectopic expression of UHRF1 or mutants. (a) DNA methylation defect in Uhrf1−/− ES cells in comparison with the wild-type E14 cells as revealed by immunofluorescent staining using anti-5-mC antibody. Also shown are the phase contrast images of the cells. Scale bar, 10 μm. (b) The Uhrf1−/− ES cells were transfected with Flag-UHRF1 or various mutants as indicated. Double immunostaining for transfected UHRF proteins was performed 3 days after transfection using a rabbit anti-Flag antibody and a mouse anti-5-mC. Also shown are the phase contrast images of the cells. The experiments were repeated at least three times for each mutant. Scale bar, 10 μm. Figure 3: Rescue of DNA methylation in Uhrf1−/− ES cells by ectopic expression of UHRF1 or mutants. ( a ) DNA methylation defect in Uhrf1−/− ES cells in comparison with the wild-type E14 cells as revealed by immunofluorescent staining using anti-5-mC antibody. Also shown are the phase contrast images of the cells. Scale bar, 10 μm. ( b ) The Uhrf1−/− ES cells were transfected with Flag-UHRF1 or various mutants as indicated. Double immunostaining for transfected UHRF proteins was performed 3 days after transfection using a rabbit anti-Flag antibody and a mouse anti-5-mC. Also shown are the phase contrast images of the cells. The experiments were repeated at least three times for each mutant. Scale bar, 10 μm. Full size image Lack of DNA methylation rescue by Tudor/SRA double mutants Having observed the rescue of DNA methylation by the Tudor mutants and the SRA mutants, we next tested the ability for the Tudor/SRA double mutants YP191/192AA+YT478/479AA and FW237/238+Y555A to rescue DNA methylation in Uhrf1−/− ES cells. In contrast to the mutants that are defective in either hemi-mCpG or H3K9me2/3-binding activity, we observed that transient expression of these mutants could not rescue the DNA methylation defect in Uhrf1−/− ES cells ( Fig. 3b ). Analysis of DNA methylation status in stable cell lines The above experiments surprisingly revealed a UHRF1-mediated DNA maintenance methylation that is not entirely dependent on its hemi-mCpG-binding activity of SRA. To validate the rescue of DNA methylation observed above, we established stable Uhrf1−/− cell lines expressing wild-type or various UHRF1 mutants. We were able to obtain cell lines that expressed wild-type UHRF1, the Tudor mutant YP191/192AA, the SRA mutants YT478/479AA and R491A, and the double mutant YP191/192AA+YT478/479AA at a level similar to that of endogenous Uhrf1 in E14 ES cells ( Fig. 4a ). We then analysed the status of DNA methylation in these stable cell lines by immunostaining. To ensure the accuracy of 5-mC immunostaining, we first generated a negative control Uhrf1−/− ES cell line that stably expresses GFP (GFP-Uhrf1−/−). The control GFP-Uhrf1−/− cells were then cocultured with various stable cells at 1:1 ratio 2 days before 5-mC immunostaining. As shown in Fig. 4b , when E14 ES cells were mixed with the GFP-Uhrf1−/− ES cells, the E14 (GFP-negative) cells were strongly stained for 5-mC, whereas the control GFP-Uhrf1−/− cells (GFP-positive) were stained negatively for 5-mC. By the same approach, we found both the UHRF1 and YP191/192AA stable cells were strongly stained for 5-mC in comparison with the control GFP-Uhrf1−/− cells ( Fig. 4b ). Furthermore, although both YT478/479AA and R491A cell lines were stained weaker than E14 and UHRF1 cells, these cells were clearly positive for 5-mC when compared with the internal control GFP-Uhrf1−/− cells. In contrast, the levels of 5-mC in the Tudor/SRA double mutant stable cells were comparable to those in GFP-Uhrf1−/− cells. These data provide compelling evidence that the hemi-mCpG-binding-deficient mutants are able to partially rescue the DNA methylation defect in Uhrf1−/− ES cells, whereas the mutant deficient in binding both hemi-mCpG and H3K9me2/3 is not. 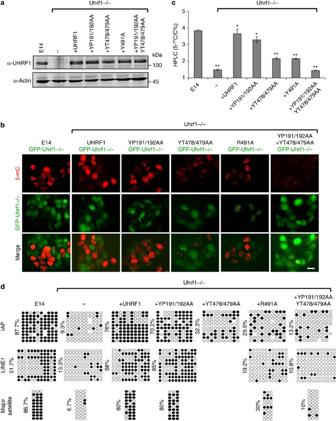Figure 4: DNA methylation status in the Uhrf1−/− ES cells stably expressing UHRF1 or mutants. (a) The selected stable Uhrf1−/− ES cell lines expressing UHRF1 or various mutants were subjected to western blot analysis using an antibody that recognizes both human UHRF1 and mouse Uhrf1. Actin served as a loading control. (b) The immunostaining analysis for 5-mC in each stable cell line was performed with a mixture of each type of stable cells and GFP-Uhrf1−/− ES cells in ~1:1 ratio. The merged images of GFP and 5-mC show that each type of stable rescue cells were stained positively for 5-mC in comparison with GFP-Uhrf1−/− ES cells except for the double mutant stable cells (YP191/192AA+YT478/479AA). Scale bar, 10 μm. (c) The genomic DNA was prepared from E14, Uhrf1−/− and each stable cell line and analysed for the levels of 5-mC by HPLC. The levels of 5-mC were shown as percentage of total cytosine. Data shown as mean±s.d. from three independent experiments. A Student’st-test was used to calculate statistical significance. *P<0.05, **P<0.01. (d) The DNA methylation status of IAP, LINE-1 and major satellite was analysed by bisulfite sequencing. The percentage of 5-mC was calculated and shown. For IAP and line-1, the differences with Uhrf1−/− were statistically significant for E14, UHRF1 and YP191/192AA (**P<0.01) and YT478/379AA and R491A (**P<0.05), but not YP191/192AA+YT478/479AA. For major satellite, the differences with Uhrf1−/− were statistically significant for E14, UHRF1 and YP191/192AA (**P<0.05), but not others. Figure 4: DNA methylation status in the Uhrf1−/− ES cells stably expressing UHRF1 or mutants. ( a ) The selected stable Uhrf1−/− ES cell lines expressing UHRF1 or various mutants were subjected to western blot analysis using an antibody that recognizes both human UHRF1 and mouse Uhrf1. Actin served as a loading control. ( b ) The immunostaining analysis for 5-mC in each stable cell line was performed with a mixture of each type of stable cells and GFP-Uhrf1−/− ES cells in ~1:1 ratio. The merged images of GFP and 5-mC show that each type of stable rescue cells were stained positively for 5-mC in comparison with GFP-Uhrf1−/− ES cells except for the double mutant stable cells (YP191/192AA+YT478/479AA). Scale bar, 10 μm. ( c ) The genomic DNA was prepared from E14, Uhrf1−/− and each stable cell line and analysed for the levels of 5-mC by HPLC. The levels of 5-mC were shown as percentage of total cytosine. Data shown as mean±s.d. from three independent experiments. A Student’s t -test was used to calculate statistical significance. * P <0.05, ** P <0.01. ( d ) The DNA methylation status of IAP, LINE-1 and major satellite was analysed by bisulfite sequencing. The percentage of 5-mC was calculated and shown. For IAP and line-1, the differences with Uhrf1−/− were statistically significant for E14, UHRF1 and YP191/192AA (** P <0.01) and YT478/379AA and R491A (** P <0.05), but not YP191/192AA+YT478/479AA. For major satellite, the differences with Uhrf1−/− were statistically significant for E14, UHRF1 and YP191/192AA (** P <0.05), but not others. Full size image Cooperation of SRA and Tudor in global DNA methylation We next determined the overall levels of DNA methylation in the stable cell lines by quantitative high-performance liquid chromatography (HPLC) analysis. In agreement with previous studies, ~4% cytosine was methylated in genomic DNA from E14 ES cells and the level of 5-mC dropped drastically to ~1.5% in the Uhrf1−/− ES cells ( Fig. 4c ). Expression of wild-type UHRF1 and Tudor mutant YP191/192AA restored the level of 5-mC to ~3.8% and 3.5%, respectively. Importantly, expression of either of the two SRA mutants increased the levels of 5-mC to ~2.3%, whereas expression of the Tudor/SRA double mutant did not lead to any increase in the level of 5-mC. We also examined the global DNA methylation status of genomic DNA derived from various stable cell lines by MspI and HpaII digestion. This analysis again revealed a differential rescue of DNA methylation in various UHRF1 stable cell lines, with the levels of DNA methylation in the order of E14≥+UHRF1≥+191/192>+478/479=+491>+191/192+478/479=Uhrf1−/− ( Supplementary Fig. S7a ). Thus, quantitative and semi-quantitative restriction digestion analyses of global DNA methylation demonstrated that loss of either hemi-mCpG or H3K9me2/3-binding activity partially impaired UHRF1-mediated DNA methylation, whereas loss of both binding activities completely abolished its function in DNA methylation. Cooperation of SRA and Tudor in gene-specific methylation Having established the effect of various UHRF1 mutants in global DNA methylation, we next examined the effect on specific genomic sequences using bisulfite sequencing analysis. We first examined DNA methylation at the promoter regions of the intracisternal A particle (IAP) and long interspersed nuclear element I (LINE-1) retrotransposons. As shown in Fig. 4d , they are strongly methylated in the E14 ES cells and become hypomethylated in the Uhrf1−/− ES cells as reported previously [13] . We found that expression of UHRF1 and YP191/192AA in Uhrf1−/− ES cells restored DNA methylation of IAP to a similar level (76% and 70.2%, respectively) as in E14 cells (87.7%) ( Fig. 4d ). Although the two SRA mutants were less efficient in restoration of DNA methylation compared with the wild-type UHRF1 and the Tudor mutant, both increased the level of DNA methylation from 9.3% in Uhrf1−/− ES cells to ~30%. Importantly, this partial rescue of DNA methylation by SRA mutants was not observed for the Tudor/SRA double mutant. Similar results were observed for LINE-1 sequences and major satellites at pericentric heterochromatin ( Fig. 4d ). We also examined the DNA methylation status in the major satellite repetitive sequences by restriction digestion with Msp1 and HpaII followed by Southern blot analysis. The results again revealed a partial rescue of DNA methylation by the SRA mutant and no rescue by the Tudor/SRA double mutant ( Supplementary Fig. S7b ). Cooperative Dnmt1 replication fork targeting by Tudor and SRA The partial rescue of DNA methylation by SRA mutants raised the question if UHRF1 associates with replication foci solely through a SRA-hemi-mCpG interaction. As reported previously [13] and shown in Fig. 5a , Dnmt1 was observed as focal staining patterns only in some of the E14 ES cells that were in mid or later S phase ( Supplementary Fig. S8 ), but not in the Uhrf1−/− cells. By immunostaining analysis of a mixed culture of the control GFP-Uhrf1−/− ES cells and individual stable cell line expressing UHRF1 or a UHRF1 mutant at 1:1 ratio, we observed restoration of Dnmt1 focal staining in the Uhrf1−/− cells expressing either wild-type UHRF1 or Tudor mutant ( Fig. 5b ). Importantly, such focal staining pattern could also be observed in the Uhrf1−/− cells expressing either of the SRA mutants YT478/479AA and R491A, but not in the cells expressing the Tudor/SRA double mutant ( Fig. 5b ). As internal control, no Dnmt1 focal staining pattern was observed in the GFP-Uhrf1−/− ES cells. Given that the DNMT1 focal staining pattern could be observed in SRA mutant but not Tudor/SRA double mutant cells, we conclude the H3K9me2/3-binding activity of UHRF1 also has a role in targeting DNMT1 to DNA replication forks. 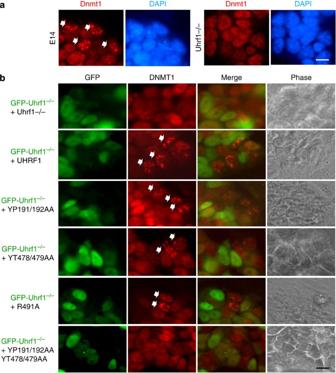Figure 5: The SRA mutants are capable of recruiting DNMT1 to DNA replication foci. (a) Loss of Dnmt1 focal staining pattern in cells replicating in mid or late S phase in Uhrf1−/− ES cells. Both E14 and Uhrf1−/− ES cells were immunostained for Dnmt1 and costained by DAPI. The cells with Dnmt1 focal staining pattern were observed only for the wild-type E14 cells. These cells were in mid or late S phase according to EdU labelling (Supplementary Fig. S7and references). Scale bar, 10 μm. (b) The immunostaining analysis for rescue of Dnmt1 focal staining pattern in each stable cell line was performed with a mixture of each type of stable cells and GFP-Uhrf1−/− ES cells in ~1:1 ratio. The representative merged images of GFP and DNMT1 show that the presence of Dnmt1 focal staining cells (marked by arrows) in comparison with the GFP-Uhrf1−/− ES cells except for the double mutant stable cells (YP191/192AA+YT478/479AA). Scale bar, 10 μm. Figure 5: The SRA mutants are capable of recruiting DNMT1 to DNA replication foci. ( a ) Loss of Dnmt1 focal staining pattern in cells replicating in mid or late S phase in Uhrf1−/− ES cells. Both E14 and Uhrf1−/− ES cells were immunostained for Dnmt1 and costained by DAPI. The cells with Dnmt1 focal staining pattern were observed only for the wild-type E14 cells. These cells were in mid or late S phase according to EdU labelling ( Supplementary Fig. S7 and references). Scale bar, 10 μm. ( b ) The immunostaining analysis for rescue of Dnmt1 focal staining pattern in each stable cell line was performed with a mixture of each type of stable cells and GFP-Uhrf1−/− ES cells in ~1:1 ratio. The representative merged images of GFP and DNMT1 show that the presence of Dnmt1 focal staining cells (marked by arrows) in comparison with the GFP-Uhrf1−/− ES cells except for the double mutant stable cells (YP191/192AA+YT478/479AA). Scale bar, 10 μm. Full size image H3K9me2/3 is required for SRA mutant-mediated DNA methylation To analyse if the partial rescue of DNA methylation by SRA mutants were indeed dependent on its H3K9me2/3-binding activity, we coexpressed UHRF1 and SRA mutants with JMJD2A (also known as KDM4A/JHDM3A), a H3K9me2/3 demethylase [34] , [35] . Pilot experiments in Fig. 6a show that expression of JMJD2A but not the enzymatic-deficient JMJD2Am mutant resulted in demethylation of H3K9me3 in Uhrf1−/− ES cells and that in co-transfection experiments most JMJD2A-expressing cells also expressed UHRF1 or mutants ( Supplementary Fig. S9 ). When co-transfected with wild-type UHRF1, we found that most of the JMJD2A or JMJD2Am-positive cells were also positive for 5-mC immunostaining ( Fig. 6b ). However, when co-transfected with the SRA R491A mutant, we observed that most of the JMJD2A-positive cells were negative for 5-mC immunostaining ( Fig. 6c ), whereas most of the JMJD2Am-positive cells were positive for 5-mC staining. Similar results were obtained when another SRA mutant YT478/479/AA was tested ( Fig. 6d ). We scored more than 200 transfected cells in three independent experiments and quantified the effect of coexpression of wild-type and mutant JMJD2A on rescue of DNA methylation by wild-type UHRF1 and SRA mutants ( Fig. 6e ). The data indicate that coexpression of JMJD2A substantially reduced the ability of the SRA mutants but not the wild-type UHRF1 to rescue DNA methylation in Uhrf1−/− ES cells, indicating that the UHRF1 SRA mutants rescue the DNA methylation defect in an H3K9me2/3-binding dependent manner. 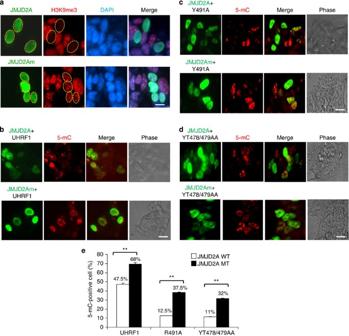Figure 6: Partial rescue of DNA methylation in Uhrf1−/− ES cells by SRA mutants requires H3K9me2/3. (a) Ectopic expression of wild-type H3K9me2/3 demethylase JMJD2A but not enzymatic defective mutant led to substantially reduced H3K9me3 in Uhrf1−/− ES cells. The cells were transfected with the Flag-JMJD2A or Flag-JMJD2Am and 2 days after transfection the cells were double immunostained with anti-Flag (green) and H3K9me3 (red) and costained with DAPI. The transfected cells were marked by circles. Scale bar, 10 μm. (b) Coexpression of Flag-JMJD2A with the wild-type UHRF1 did not affect the rescue of DNA methylation significantly. The cells were transfected with Flag-JMJD2A+UHRF1 or Flag-JMJD2Am+UHRF1 and 3 days after transfection the cells were processed for double immunostaining for Flag-JMJD2A and 5-mC. Also shown are the phase contrast images of colonies of cells. Scale bar, 10 μm. (c) and (d) The same experiments were performed with the SRA mutants R491A and YT478/479AA. Scale bar, 10 μm. (e) The quantitative results for rescue of DNA methylation in cells coexpressing Flag-JMJD2A or Flag- JMJD2Am. Data shown as mean±s.d. from three independent experiments. A Student’st-test was used to calculate statistical significance. **P<0.01. Figure 6: Partial rescue of DNA methylation in Uhrf1−/− ES cells by SRA mutants requires H3K9me2/3. ( a ) Ectopic expression of wild-type H3K9me2/3 demethylase JMJD2A but not enzymatic defective mutant led to substantially reduced H3K9me3 in Uhrf1−/− ES cells. The cells were transfected with the Flag-JMJD2A or Flag-JMJD2Am and 2 days after transfection the cells were double immunostained with anti-Flag (green) and H3K9me3 (red) and costained with DAPI. The transfected cells were marked by circles. Scale bar, 10 μm. ( b ) Coexpression of Flag-JMJD2A with the wild-type UHRF1 did not affect the rescue of DNA methylation significantly. The cells were transfected with Flag-JMJD2A+UHRF1 or Flag-JMJD2Am+UHRF1 and 3 days after transfection the cells were processed for double immunostaining for Flag-JMJD2A and 5-mC. Also shown are the phase contrast images of colonies of cells. Scale bar, 10 μm. ( c ) and ( d ) The same experiments were performed with the SRA mutants R491A and YT478/479AA. Scale bar, 10 μm. ( e ) The quantitative results for rescue of DNA methylation in cells coexpressing Flag-JMJD2A or Flag- JMJD2Am. Data shown as mean±s.d. from three independent experiments. A Student’s t -test was used to calculate statistical significance. ** P <0.01. Full size image The role of UHRF1-induced 5-mC flip out in DNA methylation A novel mechanism for binding hemi-mCpG by UHRF1 SRA domain involves 5-mC flip out of the DNA helix [18] , [19] , [20] . To test if the 5-mC flip out induced by UHRF1 is important for subsequent methylation by DNMT1, we constructed a DNMT1–PCNA fusion protein ( Fig. 7a ) and verified its expression in Uhrf1−/− ES cells upon transient transfection ( Fig. 7b ). This fusion protein is enzymatically as active as the control DNMT1 in in vitro DNA methylation assay ( Supplementary Fig. S10 ). Furthermore, in NIH3T3 cells this fusion protein, like DNMT1 and PCNA, can correctly localize to the pericentric heterochromatins in S phase of cell cycle ( Supplementary Fig. S11a ). Importantly, this PCNA–DNMT1 fusion proteins, but not the control DNMT1 localize correctly to DNA replication foci in the Uhrf1−/− ES cells ( Fig. 7c ), indicating that this fusion protein can be correctly targeted to DNA replication foci via PCNA. 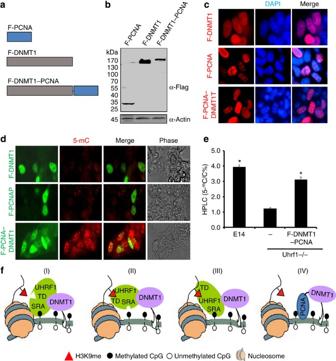Figure 7: Rescue of DNA methylation defect in Uhrf1−/− ES cells by a DNMT1–PCNA fusion protein. (a) Schematic illustration of PCNA, DNMT1 and DNMT1–PCNA fusion proteins. (b) Verification of expression of transfected PCNA, DNMT1 and DNMT1–PCNA in Uhrf1−/− ES cells. (c) Observation of focal staining pattern for DNMT1–PCNA but not DNMT1 alone. The Uhrf1−/− ES cells were transfected with the indicated expression constructs and 3 days after transfection the immunostaining for detection of Flag-tagged proteins and DAPI staining were performed. Note focal staining patterns were observed for PCNA and DNMT1–PCNA but not DNMT1 alone. Scale bar, 10 μm. (d) The Uhrf1−/− ES cells were transfected with PCNA, DNMT1 or DNMT1–PCNA and 3 days after transfection the cells were double immunostained for 5-mC and protein expression using anti-Flag antibody. Note that rescue of DNA methylation was observed only for the cells expressing DNMT1–PCNA. Scale bar, 10 μm. (e) The genomic DNA was prepared from E14, Uhrf1−/− and F-DNMT1–PCNA cell lines and analysed for the levels of 5-mC by HPLC. The levels of 5-mC were shown as percentage of total cytosine. Data shown as mean±s.d. from three independent experiments. A Student’st-test was used to calculate statistical significance. *P<0.05. (f) Working models for UHRF1-mediated recruitment of DNMT1 for DNA maintenance methylation. UHRF1 possesses both hemi-mCpG and H3K9me2/3 binding activities and can locate to replication forks through either of the binding activities (models I and II). UHRF1 is likely to bind nucleosomes with both hemi-mCpG and H3K9me2/3 marks coordinately (model III), which in turn leads to efficient recruitment of DNMT1 and DNA maintenance methylation. Furthermore, as DNMT1–PCNA fusion proteins is able to substantially rescue DNA methylation defect in Uhrf1−/− ES cells (model IV), it raises the possibility that other DNMT1-interacting proteins may have a role in targeting DNMT1 to specific genomic locus and help to maintain DNA methylation in the specific regions. MpG, hemi-mCpG; MK9, H3K9me2/3. Figure 7: Rescue of DNA methylation defect in Uhrf1−/− ES cells by a DNMT1–PCNA fusion protein. ( a ) Schematic illustration of PCNA, DNMT1 and DNMT1–PCNA fusion proteins. ( b ) Verification of expression of transfected PCNA, DNMT1 and DNMT1–PCNA in Uhrf1−/− ES cells. ( c ) Observation of focal staining pattern for DNMT1–PCNA but not DNMT1 alone. The Uhrf1−/− ES cells were transfected with the indicated expression constructs and 3 days after transfection the immunostaining for detection of Flag-tagged proteins and DAPI staining were performed. Note focal staining patterns were observed for PCNA and DNMT1–PCNA but not DNMT1 alone. Scale bar, 10 μm. ( d ) The Uhrf1−/− ES cells were transfected with PCNA, DNMT1 or DNMT1–PCNA and 3 days after transfection the cells were double immunostained for 5-mC and protein expression using anti-Flag antibody. Note that rescue of DNA methylation was observed only for the cells expressing DNMT1–PCNA. Scale bar, 10 μm. ( e ) The genomic DNA was prepared from E14, Uhrf1−/− and F-DNMT1–PCNA cell lines and analysed for the levels of 5-mC by HPLC. The levels of 5-mC were shown as percentage of total cytosine. Data shown as mean±s.d. from three independent experiments. A Student’s t -test was used to calculate statistical significance. * P <0.05. ( f ) Working models for UHRF1-mediated recruitment of DNMT1 for DNA maintenance methylation. UHRF1 possesses both hemi-mCpG and H3K9me2/3 binding activities and can locate to replication forks through either of the binding activities (models I and II). UHRF1 is likely to bind nucleosomes with both hemi-mCpG and H3K9me2/3 marks coordinately (model III), which in turn leads to efficient recruitment of DNMT1 and DNA maintenance methylation. Furthermore, as DNMT1–PCNA fusion proteins is able to substantially rescue DNA methylation defect in Uhrf1−/− ES cells (model IV), it raises the possibility that other DNMT1-interacting proteins may have a role in targeting DNMT1 to specific genomic locus and help to maintain DNA methylation in the specific regions. MpG, hemi-mCpG; MK9, H3K9me2/3. Full size image Having demonstrated the correct targeting of Flag-PCNA–DNMT1 to DNA replication foci by PCNA, we next tested the ability for this fusion protein to rescue the DNA methylation defect in Uhrf1−/− ES cells. Double immunostaining was performed to detect transfected cells using anti-Flag antibody and DNA methylation by anti−5-mC antibody. As controls, we found that expression of either Flag-DNMT1 or Flag-PCNA had no effect on DNA methylation in transfected Uhrf1−/− ES cells ( Fig. 7d ). In addition, coexpression of DNMT1 and PCNA also had no effect on DNA methylation in Uhrf1−/− ES cells ( Supplementary Fig. S11b ). However, expression of Flag-DNMT1–PCNA led to substantial increase in the levels of DNA methylation ( Fig. 7d ), indicating that targeting DNMT1 to replication forks by fused PCNA could bypass the requirement for UHRF1 in DNA maintenance methylation. To further confirm this novel finding, we also established a stable Uhrf1−/− ES cell line that expressed Flag-DNMT1–PCNA as shown by western blot analysis ( Supplementary Fig. S12a ). We carried out quantitative measurement of DNA methylation by HPLC and confirmed a substantial increase of DNA methylation in this stable cell line ( Fig. 7e ), even though immunostaining analysis revealed only ~60% cells were positive for Flag-DNMT1–PCNA ( Supplementary Fig. S12b ). In addition, analysis of global DNA methylation by HpaII digestion and Southern blot analysis of minor satellite repetitive sequences demonstrated an increase of DNA methylation in the stable cell line ( Supplementary Fig. S12c and 12d ). Considering that not all stable cells (~60%) were positive for Flag-DNMT1–PCNA, these data indicate that expression of Flag-DNMT1–PCNA in Uhrf1−/− ES led to substantial rescue of DNA methylation. As targeting DNMT1 to replication foci as a fusion protein of PCNA is able to substantially rescue DNA methylation defect in Uhrf1−/− ES cells, we conclude that the 5-mC flip out induced by binding of SRA domain of UHRF1 is unlikely to be essential for subsequent DNA methylation by DNMT1. A recent major finding in the study of DNA maintenance methylation is that UHRF1 is required for targeting DNMT1 to DNA replication forks [13] and this function of UHRF1 is conserved in evolution [36] . UHRF1 possesses a unique hemi-mCpG-binding activity, as well as a H3K9me2/3-binding activity. Given that newly replicated DNA is hemi-mCpG, this unique feature of UHRF1 provides an ideal solution for DNA maintenance methylation and have led to the working model that UHRF1 targets DNMT1 to DNA replication forks through its ability to bind hemi-mCpG and its ability to interact with DNMT1 [12] , [13] , [18] , [19] , [20] . In this study, we have dissected and systematically analysed the role of hemi-mCpG and H3K9me2/3 binding activities in UHRF1 heterochromatin association, DNMT1 replication fork targeting and DNA maintenance methylation ( Fig. 7f ). The UHRF1 mutants with loss of either hemi-mCpG or H3K9me2/3, but not both, exhibit only partial defect in heterochromatin association ( Fig. 4 ), ability to recruit Dnmt1 ( Fig. 5 ) and rescue of DNA maintenance methylation defect in Uhrf1−/− ES cells. Thus, UHRF1 is able to target DNMT1 to replication forks through independent recognition of either hemi-mCpG on nascent DNA ( Fig. 7f , model I) or H3K9me2/3 marks on the newly assembled nucleosomes ( Fig. 7f , model II). Given that a more efficient rescue of DNA methylation and DNMT1 targeting was observed for wild-type UHRF1, it is conceivable that UHRF1 makes use of both the hemi-mCpG and H3K9me2/3 binding activities to bind in a cooperative manner the nucleosomes with both hemi-mCpG and H3K9me2/3 marks ( Fig. 7f , model III), which in turn recruits DNMT1 for DNA maintenance methylation. Extensive structural studies demonstrate UHRF1 binds specifically hemi-mCpG through a novel base flip out mechanism [18] , [19] , [20] . As targeting DNMT1 to replication forks by a means of PCNA–DNMT1 fusion protein can substantially rescue DNA methylation defect in Uhrf1−/− ES cells ( Fig. 7 ), we favour the idea that the base flip out induced by SRA binding is not essential for subsequent DNA methylation by DNMT1, but serves to gain sufficient surface for specific interaction with hemi-methylated DNA. Another explanation that the base flip out by UHRF1 is likely not essential for subsequent DNA methylation is that Dnmt1 itself also has the ability to induce base flip out [37] . However, we could not rule out the possibility that the base flip induced by the binding of UHRF1 may facilitate DNA methylation by DNMT1. The ability for DNMT1–PCNA fusion to rescue DNA methylation in Uhrf1−/− ES cells also raises the possibility that other DNMT1-interacting proteins may target DNMT1 for maintaining local DNA methylation (model IV). Although our study reveals that both UHRF1 hemi-mCpG and H3K9me2/3 binding activities contribute to DNA maintenance methylation, the hemi-mCpG-binding activity appears to have a more important role in DNA maintenance methylation. By multiple assays, we showed that the Tudor mutants were more efficient in rescue of DNA methylation than the SRA mutants. In this regard, our results are not entirely consistent with a recent publication showing an essential role for UHRF1’s H3K9me2/3-binding activity in DNA maintenance methylation [38] . It is noteworthy that using Dnmt1 focal staining pattern as a mark for UHRF1-dependent replication fork targeting of Dnmt1, we showed that both types of mutants rescued Dnmt1 focal staining in Uhrf1−/− ES cells to a similar extent. Thus, the different activity in rescue of DNA methylation is likely to lie in a step downstream of Dnmt1 recruitment. However, as pointed out above, the predominant role of UHRF1’s hemi-mCpG-binding activity in DNA maintenance methylation might not be explained by a functional dependency of DNA maintenance methylation on 5-mC base flip out induced by binding of UHRF1 SRA domain. Although the exact mechanism(s) remains to be determined, it is conceivable that a functional SRA domain may allow UHRF1 to target Dnmt1 directly to hemi-mCpG sites within DNA replication forks and consequently more efficient DNA maintenance methylation. On the other hand, although UHRF1 can target Dnmt1 to replication forks in the absence of a functional SRA via its binding of H3K9me2/3, DNA methylation may be less efficient as Dnmt1 is not targeted directly to the hemi-mCpG sites. As two key mechanisms of epigenetic regulation, previous studies have revealed multiple layers of cross-talks between DNA methylation and histone methylation [37] , [39] , [40] , [41] . In this study, we demonstrate that cross-talk between H3K9 methylation and DNA methylation also occurs at the level of DNA maintenance methylation. Through a protein (UHRF1) with dual hemi-mCpG and H3K9me2/3 binding activities, DNMT1 can be targeted to DNA replication forks that are either enriched of hemi-mCpG and/or H3K9 methylated histones ( Fig. 7f , model I and II). Furthermore, the cooperative binding of chromatin through both the hemi-mCpG and H3K9me2/3 binding activities of UHRF1 provides a mechanism for high fidelity of DNA maintenance methylation and thus contribute to genome stability ( Fig. 7f , model III). Plasmids and antibodies For expression by transient transfection and by in vitro coupled transcription and translation, expression constructs for UHRF1 and various UHRF1 deletion mutants were generated by cloning the corresponding complementary DNA (cDNA) fragments generated by PCR into pSG5-Flag vector. For expression in mouse ES cells, the full-length human UHRF1 as described [21] was cloned into the pPYCAGIP vector to generate pPYCAGIP-UHRF1 with or without Flag tag. The various UHRF1 mutants (YP191/192AA, FW237/238AA, YT478/479AA, Y555A, Y491A, YP191/192AA+YT478/479AA, FW237/238AA+Y555A) in pPYCAGIP vector were then generated by PCR-directed mutagenesis. CFP-LacR-G9a was generated by cloning cDNA sequence encoding human G9a amino acids 831 to 1210 (the C-terminus) into PECFPC1 vector. The CFP-LacR-G9a mutant was created by introducing a point mutation (H1113K) using PCR-directed mutagenesis. pCDNA3.1-Flag-JMJD2A and its enzymatic inactive mutant were as described [28] . For expressing Flag-PCNA or Flag-DNMT1 in ES cells, the full-length cDNA for PCNA or DNMT1 was cloned into the pPYCAGIP-Flag vector. The pPYCAGIP-Flag-DNMT1–PCNA plasmid was generated by inserting the coding region of PCNA downstream of DNMT1 in the pPYCAGIP-Flag-DNMT1. For expression of UHRF1 SRA domain as a GST-fusion protein, the cDNA fragment encoding UHRF1 amino acids 386–650 was cloned into pGEX4T-1 and derivative SRA mutants (YT478/479, Y555A and R491A) were then generated by PCR-directed mutagenesis. All plasmids were verified by DNA sequencing. The antibodies used included UHRF1(AbMART), H3K9me3 (Abcam), DNMT1 (AbMART), Flag (Sigma-Aldrich), Flag (HuaAn corporation ) and methyl-C (Eurogentec). Cell culture, transient transfection and immunofluorescence staining NIH3T3, HeLa and 293T cells were routinely maintained with regular DMEM plus 10% FBS (GIBCO). E14 and mUhrf1-/ ESCs were cultured on mouse embryonic fibroblast feeder cells in DMEM supplemented with 10% FBS, 1000, units ml −1 leukaemia inhibitory factor, 50 U ml −1 penicillin and 50 mg ml −1 streptomycin, X1 non-essential amino acids, 1 mM sodium pyruvate, 2 mM L -glutamine and 55 μM beta-mercaptoethanol (Sigma-Aldrich). Transient transfections of NIH3T3, DG44-CHO and UHRF1−/− ES cells were carried out using Lipofectamine 2000 (Invitrogen) essentially according to the manufacturer’s instruction. For immunofluorescence staining of 5-meC and DNMT1, NIH3T3 or Uhrf1−/− ES cells were washed with X1 PBS (137 mM NaCl, 2.7 mM KCl, 10 mM Na 2 HPO 4 and 2 mM KH 2 PO 4 ) prior to fixation in 4% paraformaldehyde. Cells for 5-mC immunostaining were incubated with 4 N HCl at room temperature for 30 min, whereas the cells for DNMT1 immunostaining were incubated with 1 N HCl on ice for 10 min and 2 N HCl at 37 °C for 10 min once again. The cells then neutralized with sodium borate (pH 9.0) at room temperature for 20–30 min, blocked with 5% BSA in 37 °C incubator for 15–20 min and incubated with 5-meC or DNMT1 antibody for 2 h or overnight. For double immunostaining with 5-mC, the cells were treated as for 5-mC immunostaining and then incubated with both primary antibodies (one mouse monoclonal antibody and the other rabbit polyclonal antibody), followed by incubation with Alexa Fluor 488 and Texas-Red-conjugated secondary antibodies against mouse or rabbit primary antibodies. Images were acquired with an Olympus TH4-20D microscope system. For examining co-localization in DG44-CHO cells, Lac-CFP or Lac-CFP-G9a or Lac-CFP-G9am were co-transfected with Flag-UHRF1 or UHRF1 mutant as indicated into DG44-CHO cells. One day after transfection, cells were processed for immunostaining using anti-Flag antibody for UHRF1. The images were acquired and examined for co-localization of CFP-Lac-G9a or G9am fusion proteins with the Flag-tagged protein of interest. For comparison of 5-mC and DNMT1 localization in the UHRF1 rescued Uhrf1−/− ES cell lines with an internal control GFP-Uhrf1−/− ES cell line, the 1:1 mixture of the each UHRF1 rescued line of cells and GFP-Uhrf1−/− ES cells were grown on glass coverslips. The immunostaining for 5-mC or DNMT1 was then performed as above. In vitro binding of histone tail peptides with 35 S-methionine-labelled proteins The assay for binding of UHRF1 and mutants to synthetic H3 tail peptide by pulldown was essentially as described [21] . Briefly, for defining H3K9me2/3-binding domain of UHRF1, various 35S-methionine-labelled UHRF1 deletion or point mutation mutants were generated with the Transcription and translation coupled reticulocyte lysate system (Promega). Biotinylated histone H3 tail peptides were synthesized and purified by Beijing Scilight Biotechnology LLC. Approximately 1 μg of different histone H3 tail (aa1-21) peptides immobilized on streptavidin-coated beads were incubated with 1:10 diluted radiolabeled proteins in binding buffer (20 mM HEPES (pH 7.9), 150 mM KCl, 1 mM dithiothreitol (DTT), 1 mM phenylmethyl sulphonyl fluoride, 10% glycerol, 0.1% NP-40 and proteinase inhibitors) for 3 h at 4 °C. The unbound proteins were removed by washing the beads four times, 5 min each, with washing buffer (20 mM HEPES (pH 7.9), 150 mM KCl, 1 mM DTT, 1 mM phenylmethyl sulphonyl fluoride, 0.1% NP-40, proteinase inhibitors). The proteins bound to the peptides were boiled in X1 SDS loading buffer and analysed by SDS–PAGE followed by autoradiography. Gel mobility shift assay The binding of hemi-methylated DNA by recombinant UHRF1 SRA domains or full-length UHRF1 proteins using gel mobility shift was essentially as described [42] . Briefly, the recombinant GST–SRA fusion proteins (wild-type and mutants) were expressed and purified from Escherichia coli using GST-glutathione beads essentially according to the manufacturer’s instruction. For testing their hemi-mCpG binding activities, ~2.5 μg recombinant GST–SRA fusion proteins were incubated with 32p-labelled hemi-mCpG probes in the binding buffer (10 mM Tris-Cl, pH 7.5, 50 mM NaCl, 5 mM MgCl2, 1 mM DTT, 0.05% NP-40, 5% glycerol, 50 ng/ μl −1 poly(dI-dC)) at room temperature for 40 min. The reactions were then electrophoresed on a 5% polyacrylamide gel in X0.5 TBE buffer at 100 V for 0.5 h. The results were visualized through autoradiography. For testing the hemi-mCpG binding activities of various SRA mutants in the context of full-length proteins, the full-length UHRF1 and SRA mutants were produced by in vitro coupled transcription and translation and then subjected to gel mobility shift assay as above. The sequences of forward and reverse strands of hemi-mCpG probe are 5′-AGCTG C G C GCAAT C GAT C GC C GGA C GT-3′, 5′-GATCACGTCCGGCGATCGATTGCGCGC-3′, in which the positions of methyl-C were underlined. Analysis of DNA Methylation by HPLC, restriction digestion and Southern blot analysis Various UHRF1 rescued Uhrf1−/− ES lines of cells were resuspended with lysis buffer (10 mM Tris-Cl (pH 7.5), 10 mM EDTA, 10 mM NaCl, 0.5% sarcosyl, 1 mg ml −1 Proteinase K) and incubated at 60 °C overnight. Then, genomic DNA was extracted by phenol/chloroform and ethanol precipitated. The samples were resuspended in TE buffer and RNaseA and RNaseH1 were added to a final concentration of 0.1 μg μl −1 and 2 U μl −1 , respectively. The RNA-free genomic DNAs were obtained by phenol/chloroform extraction followed by ethanol precipitation. Ten micrograms of genomic DNA were incubated overnight in 50 μl of the hydrolysis solution (20 mM NaAc (pH 5.3), 1 mM ZnSO 4 , 10 U ml −1 nuclease P1 (Sigma)) at 37 °C and 10 U CIP(NEB) was then added and incubated for additional 2 h at 37 °C. Twenty microliters of hydrolyzate were analysed using a HPLC system (Agilent Technologies, 1200 Series), equipped with an Agilent Eclipse XDB-C18 column (5 μm, 4.6 × 250 mm, Agilent Technologies Inc.). Detector was set-up for 280 nm and the peaks of 2′-Deoxycytidine-5′-Monophosphate and 5′-me-dCMP were confirmed by comparison of peaks with different combinations of dCMP and 5′-me-dCMP standard (Hongene Biotechnology Ltd). The restriction digestion and subsequent Southern blot analysis were performed as described [13] . Bisulfite sequencing To prepare genomic DNA, cells were lysed with the lysis buffer (10 mM Tris-Cl (pH 7.5), 10 mM EDTA, 10 mM NaCl, 0.5% sarcosy, 1 mg ml −1 Proteinase K) and incubated overnight at 60 °C. The cell lysates were extracted with phenol–chloroform once, followed by one extraction with chloroform, and genomic DNAs were ethanol precipitated. Bisulfite conversion was performed using the EpiTect Bisulfite Kit (Qiagen) according to the manufacturer’s protocol. Bisulfite-treated DNA was used to amplify, amplified regions were cloned into pEASYT1(TransGen Biotech) and sequenced. The primers for PCR amplification of IAP, LINE-1 and major satellite sequences are as follow: 5′-GGAATATGGTAAGAAAATTGAAAATTATGG-3′ and 5′-CCATATTCCAAATCCTTCAATATACATTTC-3′ for major satellite; 5′-TAGGAAATTAGTTTGAATAGGTGAGAGGT-3′ and 5′-TCAAACACTATATTACTTTAACAATTCCCA-3′ for Line-1; 5′-TTGTGTTTTAAGTGGTAAATAAATAATTTG-3′and 5′-AAAACACCACAAACCAAAATCTTCTAC-3′ for IAP. How to cite this article: Liu, X. et al . UHRF1 targets DNMT1 for DNA methylation through cooperative binding of hemi-methylated DNA and methylated H3K9. Nat. Commun. 4:1563 doi: 10.1038/ncomms2562 (2013).